Dinosaur morphological diversity and the end-Cretaceous extinction The extinction of non-avian dinosaurs 65 million years ago is a perpetual topic of fascination, and lasting debate has focused on whether dinosaur biodiversity was in decline before end-Cretaceous volcanism and bolide impact. Here we calculate the morphological disparity (anatomical variability) exhibited by seven major dinosaur subgroups during the latest Cretaceous, at both global and regional scales. Our results demonstrate both geographic and clade-specific heterogeneity. Large-bodied bulk-feeding herbivores (ceratopsids and hadrosauroids) and some North American taxa declined in disparity during the final two stages of the Cretaceous, whereas carnivorous dinosaurs, mid-sized herbivores, and some Asian taxa did not. Late Cretaceous dinosaur evolution, therefore, was complex: there was no universal biodiversity trend and the intensively studied North American record may reveal primarily local patterns. At least some dinosaur groups, however, did endure long-term declines in morphological variability before their extinction. Few issues in the history of palaeontology have fuelled as much research and popular fascination as the extinction of non-avian dinosaurs at the end of the Cretaceous (65.5 Myr ago) [1] , [2] , [3] . Despite 30 years of intensive research, a fundamental question remains: were dinosaurs undergoing a long-term decline before intensive volcanism and the Chicxulub bolide impact in the latest Cretaceous, or did these contingencies of Earth history strike down dinosaurs during or near their prime (at a time when their global biodiversity was stable or even increasing) [3] , [4] , [5] , [6] , [7] , [8] , [9] , [10] , [11] , [12] , [13] , [14] , [15] ? Previous work has focused almost exclusively on trends in taxonomic diversity (raw counts of species or genus richness) and absolute faunal abundance of dinosaurs during the final 20 million years of the Cretaceous. Diversity counts, however, are problematic because of the emerging realizations that observed taxonomic richness is heavily biased by uneven sampling of the fossil record [16] , [17] and that many supposed Late Cretaceous dinosaur species are likely juveniles or sexual morphs of other known taxa [18] , [19] , [20] . Attempts to 'correct' terminal Cretaceous diversity counts for such biases have produced conflicting results [10] , [11] , [12] , [13] , [14] , [15] . Similarly, abundance measures are also potentially distorted by taphonomic and palaeoenvironmental heterogeneity over time [21] . Finally, understanding the global picture of Late Cretaceous dinosaur evolution may be complicated by a traditional focus on the North American record [22] , particularly the abundance and distribution of dinosaurs within a single formation (Hell Creek Formation). This is understandable, as the Hell Creek is one of the few units that globally preserves a dinosaur-dominated ecosystem and a precisely located Cretaceous–Palaeogene boundary [4] , [5] , [6] , [7] , [8] , but may be only partially informative, if there were region-specific trends in biodiversity. It also cannot reveal patterns that occurred over longer timescales (for example, the last 12 million years of the Cretaceous). Quantitative analysis of morphological disparity—the variability in anatomical characters and body plans expressed by a group of organisms [23] , [24] , [25] , [26] , [27] —can also provide crucial insights into the evolutionary trajectory of dinosaurs during the latest Cretaceous. Disparity measures document changes in the anatomical diversity of clades, which may be a general proxy for the breadth of functional and ecological behaviour expressed, regardless of whether those clades had high or low species richness or faunal abundance. Variance-based disparity measures also have the benefit of being relatively robust to uneven sampling over time [23] , [24] , whereas range-based metrics are robust to disagreements in taxonomic lumping and splitting [23] (see Supplementary Text ). We suggest, therefore, that disparity may have some key advantages over species richness and abundance metrics for assessing long-term declines, increases, or plateaus in biodiversity, as it is theoretically less biased by sampling, and may better represent the spectrum of body plans, behaviours, and ecological niches exploited by a group. Disparity does not make richness and abundance data obsolete, but is an alternative biodiversity metric with its own insight and advantages. Crucially, it is a virtually untapped metric for understanding Late Cretaceous dinosaur biodiversity dynamics and promises to reveal new insights into the end-Cretaceous dinosaur extinction. We calculated four measures of range and variance-based disparity for seven major Late Cretaceous non-avian dinosaur groups [28] , [29] , [30] , [31] , [32] , [33] , [34] , to test whether disparity increased, decreased, or stayed consistent during the final two stages of the Cretaceous (Campanian and Maastrichtian). Taxa were temporally binned using two schemes (equal-length late Campanian and Maastrichtian bins ( Fig. 1 ), and three equal-length bins spanning the terminal 12 million years of the Cretaceous for North American taxa ( Fig. 2 )), and, when possible, disparity was calculated both globally and locally (for North America and Asia). Our results demonstrate both geographic and clade-specific heterogeneity in dinosaur disparity trends, and indicate that Late Cretaceous dinosaur evolution and extinction were complex. 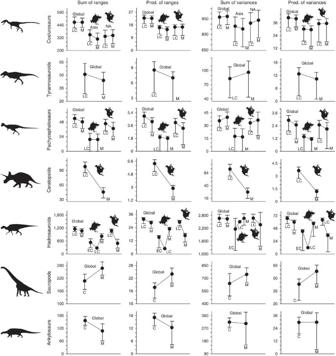Figure 1: Late Campanian and Maastrichtian disparity trends in seven dinosaur clades on global and regional scales. Four disparity metrics are shown (sum of ranges, product of ranges, sum of variances, product of variances on principal component axes representing overall morphology). Each plot contains either one or three sets of comparisons between late Campanian (LC) and Maastrichtian (M) disparity values (Asian hadrosauroids are also subdivided into a further Early Cretaceous bin (EC) whereas sauropods and ankylosaurs are binned at the coarser Campanian level (C)). For tyrannosauroids, sauropods, and ankylosaurs only global disparity measures are presented, but for coelurosaurs, pachycephalosaurs, and hadrosauroids, the disparity of global, Asian, and North American taxon sets are shown, whereas, for ceratopsids, the disparity of only North American taxa are shown. Whiskers represent the extent of 95% error bars. Statistical significance of disparity comparisons is indicated by the non-overlap of error bars. Silhouettes courtesy of Scott Hartman (http://www.skeletaldrawing.com/). Figure 1: Late Campanian and Maastrichtian disparity trends in seven dinosaur clades on global and regional scales. Four disparity metrics are shown (sum of ranges, product of ranges, sum of variances, product of variances on principal component axes representing overall morphology). Each plot contains either one or three sets of comparisons between late Campanian (LC) and Maastrichtian (M) disparity values (Asian hadrosauroids are also subdivided into a further Early Cretaceous bin (EC) whereas sauropods and ankylosaurs are binned at the coarser Campanian level (C)). For tyrannosauroids, sauropods, and ankylosaurs only global disparity measures are presented, but for coelurosaurs, pachycephalosaurs, and hadrosauroids, the disparity of global, Asian, and North American taxon sets are shown, whereas, for ceratopsids, the disparity of only North American taxa are shown. Whiskers represent the extent of 95% error bars. Statistical significance of disparity comparisons is indicated by the non-overlap of error bars. Silhouettes courtesy of Scott Hartman ( http://www.skeletaldrawing.com/ ). 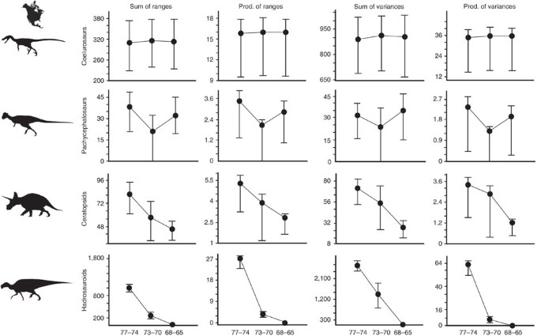Figure 2: Disparity trends across the final 12 million years of the Cretaceous for North American members of four dinosaur clades. Four disparity metrics are shown (sum of ranges, product of ranges, sum of variances, product of variances on principal component axes representing overall morphology). Each plot contains disparity values for three approximately equal-length time bins (77–74 Myr ago, 73–70 Myr ago, 68–65 Myr ago). Full size image Figure 2: Disparity trends across the final 12 million years of the Cretaceous for North American members of four dinosaur clades. Four disparity metrics are shown (sum of ranges, product of ranges, sum of variances, product of variances on principal component axes representing overall morphology). Each plot contains disparity values for three approximately equal-length time bins (77–74 Myr ago, 73–70 Myr ago, 68–65 Myr ago). Full size image Subgroup and regional disparity trends Non-avian coelurosaurs, tyrannosauroids, pachycephalosaurs, and ankylosaurs exhibit no significant changes in disparity during the late Campanian and Maastrichtian, both locally and (where measurable) globally ( Figs 1 and 2 ). Sauropods exhibit a nonsignificant increase between the Campanian and Maastrichtian in all disparity metrics, but some of these comparisons (range metrics) approach significance. In contrast, ceratopsids, all of which are North American in our dataset, exhibit significant decreases between the late Campanian and Maastrichtian in all four disparity metrics ( Fig. 1 ). Furthermore, in the three-bin North American analysis, ceratopsids exhibit a general trend of decreasing disparity, with a significant decline between the early late Campanian and latest Maastrichtian ( Fig. 2 ). We note here that this decline was likely more severe than indicated by our disparity metrics. Because centrosaurines (only a few of which are included in our dataset) exhibited considerable diversity in the Campanian, but are as yet unknown in the Maastrichtian, the inclusion of additional centrosaurine taxa would only serve to increase the already significant disparity difference between the Campanian and Maastrichtian (and sub-bins). Hadrosauroids exhibit nonsignificant decreases in global disparity between the late Campanian and Maastrichtian in all four metrics ( Fig. 1 ). There is a regional disconnect, however, because North American hadrosauroids exhibit a decrease on all metrics (significant for three of the four metrics, although not sum of variances) whereas Asian taxa exhibit nonsignificant increases on all metrics. The North American decline is starkly illustrated by the three-bin analysis, which shows a trend of decreasing disparity across the final 12 million years of the Cretaceous, including significant decreases between successive time bins for all metrics ( Fig. 2 ). A similar result of decreasing Late Cretaceous disparity in North American hadrosaurids (one subgroup of hadrosauroids) was recently reported using geometric morphometric proxies for skull shape [35] , and the congruence between this study and our analysis (using discrete characters) suggests that the disparity decline is robust. Subsampling and sample-size bias In the above disparity comparisons, sample sizes between time bins are often unequal. This may, in some cases, artificially inflate disparity values in better sampled bins relative to poorer sampled bins. Variance-based disparity metrics are relatively robust to this bias, but range-based metrics can be especially susceptible [23] , [24] . Therefore, it is important to use a subsampling technique like rarefaction to simulate equal sampling between bins ( Figs 3 and 4 ). 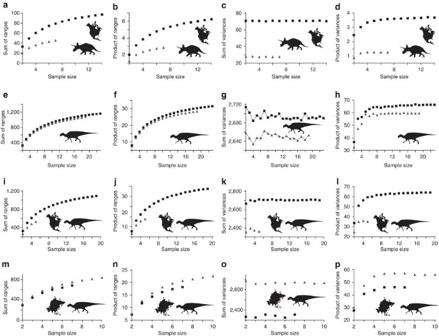Figure 3: Disparity comparisons between late Campanian and Maastrichtian time bins affected by uneven sample size. Rarefaction plots showing how disparity comparisons between late Campanian and Maastrichtian time bins (Fig. 1) are affected by uneven sample size. (a–d) North American ceratopsids. (e–h) Global hadrosauroids. (i–l) North American hadrosauroids. (m–p) Asian hadrosauroids. Each plot shows the disparity value of a certain group (for example, late Campanian ceratopsids) calculated at ever smaller subsampled sample sizes, which permits comparison of disparity between late Campanian and Maastrichtian groups at equal sample sizes. For each set of taxa, all four disparity metrics are shown. Triangles refer to Maastrichtian values and squares late Campanian values (for Asian hadrosauroids early and late Campanian values are pooled). The late Campanian–Maastrichtian disparity decrease for global ceratopsids, global hadrosauroids, and North American hadrosauroids is found whenever sample sizes are equalized, down to a common size of two taxa in both time bins. Although nonsignificant (Fig. 1), the Campanian–Maastrichtian disparity increase exhibited by Asian hadrosauroids is also seen whenever sample sizes are equalized, lending credence to the hypothesis that there was a true disparity increase. Figure 3: Disparity comparisons between late Campanian and Maastrichtian time bins affected by uneven sample size. Rarefaction plots showing how disparity comparisons between late Campanian and Maastrichtian time bins ( Fig. 1 ) are affected by uneven sample size. ( a – d ) North American ceratopsids. ( e – h ) Global hadrosauroids. ( i – l ) North American hadrosauroids. ( m – p ) Asian hadrosauroids. Each plot shows the disparity value of a certain group (for example, late Campanian ceratopsids) calculated at ever smaller subsampled sample sizes, which permits comparison of disparity between late Campanian and Maastrichtian groups at equal sample sizes. For each set of taxa, all four disparity metrics are shown. Triangles refer to Maastrichtian values and squares late Campanian values (for Asian hadrosauroids early and late Campanian values are pooled). The late Campanian–Maastrichtian disparity decrease for global ceratopsids, global hadrosauroids, and North American hadrosauroids is found whenever sample sizes are equalized, down to a common size of two taxa in both time bins. Although nonsignificant ( Fig. 1 ), the Campanian–Maastrichtian disparity increase exhibited by Asian hadrosauroids is also seen whenever sample sizes are equalized, lending credence to the hypothesis that there was a true disparity increase. 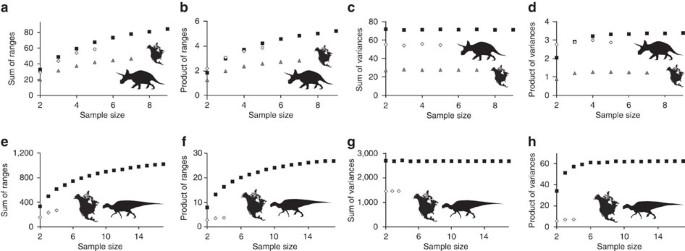Figure 4: Disparity comparisons between three equal-length latest Cretaceous time bins affected by uneven sample size. Rarefaction plots showing how disparity comparisons between three equal-length latest Cretaceous time bins (Fig. 2) are affected by uneven sample size. (a–d) North American ceratopsids. (e–h) North American hadrosauroids. Squares refer to 77–74 Myr ago values, diamonds 73–70 Myr ago values, and triangles 68–65 Myr ago values. The general disparity decrease across all three bins for ceratopsids is recovered at all sample sizes down to a common size of four, whereas the significant decrease between 77–74 Myr ago and 68–65 Myr ago disparity is seen at all sample sizes. The significant decrease between 77–74 and 73–70 hadrosauroid disparity is seen at all sample sizes (68–65 Myr ago hadrosauroid values not shown here, because there is only a single taxon in this bin and therefore disparity is always at zero). Full size image Figure 4: Disparity comparisons between three equal-length latest Cretaceous time bins affected by uneven sample size. Rarefaction plots showing how disparity comparisons between three equal-length latest Cretaceous time bins ( Fig. 2 ) are affected by uneven sample size. ( a – d ) North American ceratopsids. ( e – h ) North American hadrosauroids. Squares refer to 77–74 Myr ago values, diamonds 73–70 Myr ago values, and triangles 68–65 Myr ago values. The general disparity decrease across all three bins for ceratopsids is recovered at all sample sizes down to a common size of four, whereas the significant decrease between 77–74 Myr ago and 68–65 Myr ago disparity is seen at all sample sizes. The significant decrease between 77–74 and 73–70 hadrosauroid disparity is seen at all sample sizes (68–65 Myr ago hadrosauroid values not shown here, because there is only a single taxon in this bin and therefore disparity is always at zero). Full size image Rarefaction indicates that all of the above mentioned statistically significant disparity comparisons show consistent patterns of increase or decrease when samples are reduced and equalized down to a small common sample size of taxa in all analysed Campanian and Maastrichtian bins ( Figs 3 and 4 ). These include the late Campanian–Maastrichtian decrease for ceratopsids on all four metrics (down to a common sample size of two), the 77–74 Myr ago to 68–65 Myr ago decrease for North American ceratopsids (common sample size of four), the late Campanian–Maastrichtian decrease for North American hadrosauroids based on the two range metrics and product of variances (common sample size of two), and the 77–74 Myr ago to 73–70 Myr ago to 68–65 Myr ago decrease for North American hadrosauroids on all four metrics (common sample size of two). Additionally, rarefaction helps to interpret some disparity comparisons that seem marked but were determined as nonsignificant, most likely because of small sample sizes in some bins (which increase the size of error bars, making it more likely that error bars overlap and render a comparison nonsignificant). On all four disparity metrics, Asian Maastrichtian hadrosauroids have greater disparity than Campanian taxa when sample sizes are equalized between the two bins, down to a common sample size of two ( Fig. 3 ). Additionally, the nonsignificant decrease in global hadrosauroid disparity between the late Campanian and Maastrichtian, which is seen on all four metrics, is maintained in each case when both time bins are rarefied down to a common sample size of two ( Fig. 3 ). Finally, the increase in global sauropod disparity between the Campanian and Maastrichtian, also present but nonsignificant on all four metrics, is maintained in each case, when both bins are rarefied to a common sample of two taxa ( Supplementary Fig. S1 ). Although rarefaction is not immune to biases relating to differences in original sample size [24] , these results do lend credence to the interpretations that Asian hadrosauroids increased in disparity during the latest Cretaceous, global hadrosauroids declined in disparity, and global sauropods increased in disparity. Compared with most previous studies that focused on species richness or faunal abundance, these disparity calculations paint a more nuanced picture of the final 12 million years of dinosaur history. The most salient result is that trends in Campanian–Maastrichtian disparity are heterogeneous, with different clades and geographic regions showing different patterns. Some clades maintain consistent disparity across the late Campanian and Maastrichtian, most notably the carnivorous theropod dinosaurs (Coelurosauria, Tyrannosauroidea) and the small-to-medium-sized herbivorous pachycephalosaurs and ankylosaurs. One group, the enormous bulk-feeding sauropods (which did not have advanced chewing abilities), may have undergone a Campanian–Maastrichtian disparity increase, judging by the rarefaction results. On the other hand, the two clades of large-bodied, bulk-feeding herbivores with sophisticated jaw occlusion and dental batteries (Hadrosauroidea, Ceratopsidae) exhibit marked decreases. This suggests that there are not only clade-specific disparity patterns, but also that different ecological categories of dinosaurs (differing in diet and body size) may have experienced distinct macroevolutionary trajectories during the Late Cretaceous. A strict interpretation of the results suggests that large-bodied herbivores with advanced shearing abilities may have experienced a terminal Cretaceous decline, whereas smaller herbivores, enormous herbivores without advanced chewing abilities, and carnivorous dinosaurs remained relatively stable (or even increased in disparity) over this time. Intriguingly, a recent survey of dinosaur species richness during the terminal Cretaceous recovered global trends broadly similar to our disparity results: static theropod diversity, a marked ornithischian decrease likely driven largely by loss of hadrosauroid and ceratopsian species, and an increase in sauropod diversity [15] The broad congruence between species richness and disparity suggests that both metrics are converging on a common pattern (see also ref. 11 ). What is clear from both disparity and species richness studies, at the very least, is that there is not a single overarching trend characteristic of all non-avian dinosaurs. It is also evident that some clades experienced dissimilar, and even opposite, disparity trajectories in different geographic regions. The prime example is hadrosauroids, which underwent a significant late Campanian–Maastrichtian disparity decrease in North America but a possible increase in Asia (which, although insignificant, is consistently found when all four metrics are subject to rarefaction). Almost all work on Late Cretaceous dinosaur diversity and abundance has focused either on pooled global datasets or the North American record, which is understandable given the relatively limited number of quality Campanian–Maastrichtian dinosaur fossils from other continents and the detailed stratigraphic understanding of the well-sampled Hell Creek Formation [4] , [5] , [6] , [7] , [8] . It may be, however, that the North American record represents a local anomaly. Extreme fluctuations of the inland Western Interior Sea, mountain building, and proposed biogeographic provincialism [31] may have affected the evolution of North American dinosaurs in distinct ways from species on other continents, meaning that the North American record may not be representative of a global pattern, if one exists. A renaissance in the discovery of Cretaceous Asian dinosaurs over the past two decades has enabled our calculations of separate disparity measures for Asian species, and future work should focus on Asia-specific diversity and abundance trends like those widely compiled and debated for North American dinosaurs [15] . In sum, disparity trends indicate that Late Cretaceous dinosaur evolution was complex. Overall variability in dinosaur morphology was both clade and region-specific. A similar pattern of regional and subclade variability is also apparent in species richness data [11] , [15] , which further reinforces the hypothesis that terminal Cretaceous dinosaur evolution was not globally uniform. This raises the likelihood that pooled global diversity datasets may mask distinct regional trends, and that focus on the North American record (both regarding diversity and abundance) may primarily reveal local patterns. Our disparity results do not provide support for a universal decline, plateau, or increase in terminal Cretaceous dinosaur biodiversity. Some clades (ceratopsids, hadrosauroids), ecological types (large-bodied bulk-feeding herbivores with sophisticated feeding mechanisms), and geographic groupings (some North American taxa) underwent a disparity decrease during the late Campanian–Maastrichtian. Others, however, including carnivorous dinosaurs, mid-sized herbivores, and some Asian taxa evidently did not. It must be remembered that our coarse time bins, which are necessary because of the imprecise ages of most fossils included in our study [12] , only examine changes between two or three subintervals of the latest Cretaceous, and results will likely be refined as the temporal ages of fossils become better constrained [10] . It should also be remembered that, whatever the cause and tempo of the dinosaur extinction, by the beginning of the Paleocene non-avian dinosaur disparity was zero, indicating that the focal point of the extinction was within or at the end of the Maastrichtian, the final bin in our analysis. Even if the disparity of some dinosaur clades or regional faunas were in decline during the terminal Cretaceous, this does not automatically mean that dinosaurs were doomed to extinction. Dinosaur disparity and diversity fluctuated throughout the Mesozoic [11] , [12] , [15] , [36] , [37] , and small increases or decreases between two or three time intervals (such as the late Campanian and Maastrichtian) may not be noteworthy within the context of the entire 150+-million-year history of the clade. Unfortunately, records of dinosaur disparity across the entire Mesozoic are not yet available for comparison, and are difficult to compile because of low sample sizes in many stage-level intervals, but the establishment of these patterns should be a major goal of research on dinosaur biodiversity. Furthermore, there are known instances in the fossil record in which major vertebrate clades endured catastrophic diversity and disparity losses, both during mass extinctions and normal background times, but later rebounded [36] , [37] , [38] , [39] , [40] . A satisfactory understanding of the causes and tempo of the non-avian dinosaur extinction remains difficult, but the compilation of additional biodiversity metrics (such as disparity) and increased study of non-North American taxa is helping to bring clarity. Groups analysed We calculated the terminal Cretaceous disparity patterns of every dinosaur subgroup that is represented by a reasonable number of Campanian–Maastrichtian specimens that could be scored for large matrices of discrete characters. Analysed clades include: non-avian coelurosaurian theropods [28] , tyrannosauroid theropods [29] , pachycephalosaurs [30] , ceratopsids (most of which are chasmosaurines, because there is no available global phylogeny of ceratopsids that includes comprehensive sampling of centrosaurines and chasmosaurines [31] ), hadrosauroids [32] , sauropods [33] , and ankylosaurs [34] . Other groups, such as abelisauroid theropods, non-hadrosauroid ornithopods, and non-ceratopsid ceratopsians, could not be analysed because large samples of reasonably complete Campanian–Maastrichtian specimens scored for discrete character data are not yet available, almost entirely due to poor fossil sampling [41] , [42] , [43] . Birds were not included in the coelurosaur dataset, because we chose to focus specifically on non-avian dinosaurs, and more importantly, because of severe sampling biases that limit the number of Maastrichtian specimens that can be scored for large numbers of discrete characters [44] , [45] . We included as many specimens as possible in each of the seven analysed datasets, but, because of long-standing historical collection biases, there is an abundance of Laurasian (North American and Asian) taxa relative to Gondwanan taxa in all datasets, with the exception of sauropods. It is possible, therefore, that our results are mostly applicable to Laurasia and might not reveal truly global disparity patterns. All taxa included in the analyses, along with their temporal and provenance information, are listed in Supplementary Table S1 . Disparity calculations The seven discrete character datasets record the presence, absence, number, and form of skeletal features in each species of the clade being analysed, and, therefore, comprise a database of overall morphological form for the group. Each of the seven discrete character datasets [28] , [29] , [30] , [31] , [32] , [33] , [34] was used to derive a Euclidean distance matrix, which quantifies the pairwise differences between the taxa in question, using the freeware program MATRIX. The seven distance matrices were next subjected to individual principal coordinates analyses (PCO), a multivariate statistical technique that assimilates information from the distance matrix into a more manageable set of coordinate axes, using the freeware program GINGKO (Universitat de Barcelona, http://biodiver.bio.ub.es/ginkgo/ ). The first axis represents those character distances contributing most to the overall variability among species, and each additional axis represents distances of progressively less significance. The seven PCO analyses returned sets of PCO scores for each species on each PCO axis, which together represent proxies for the overall form of each taxon ( Supplementary Table S2 ). Four disparity metrics were calculated for each set of species in each time bin: the sum and product of the ranges and the variances on the set of PCO axes that together described 90% of total variance. The number of axes used for each clade is as follows: coelurosaurs (20), tyrannosauroids (6), pachycephalosaurs (11), ceratopsids (15), hadrosauroids (37), sauropods (11), and ankylosaurs (9). The disparity metrics were calculated using the software program RARE [46] , and the two multiplicative metrics were normalized by taking the root corresponding to the number of PCO axes used (for example, in the case of coelurosaurs, they were normalized by taking the twentieth root). Range measures quantify the entire spread of morphological variation exhibited by the set of taxa in question, whereas variance measures describe the mean dissimilarity among forms (the spread of taxa in morphospace). The statistical significance of two disparity comparisons was assessed by the overlap (nonsignificant) or non-overlap (significant) of 95% confidence intervals, generated by bootstrapping in RARE (1,000 replicates). Rarefaction was also performed in RARE, to compensate for unequal sample sizes between bins. Taxon age binning Taxon ages were determined using the Palaeobiology Database (paleodb.org/). Because the Paleobiology Database also includes records of fragmentary specimens that have been assigned to a certain species in the literature (sometimes, regardless of whether or not that assignment is well-argued or based on firm evidence), we scrutinized each relevant entry and only considered specimens that could confidently be assigned to a species using apomorphies. Taxa were then binned into temporal categories using two approaches. First, all taxa in the seven clades were placed in approximately equal-length late Campanian (77–70.5 Myr ago) and Maastrichtian (70.5–65 Myr ago) bins. Because of low sample sizes, all known Campanian sauropods and ankylosaurs that could be scored for the discrete character datasets were included in the late Campanian bin. Coelurosaurs, pachycephalosaurs, and hadrosauroids were analysed both globally and locally (separate bins for North American and Asian taxa), but tyrannosauroids, sauropods, and ankylosaurs could only be analysed globally owing to small regional sample sizes, whereas ceratopsids could only be analysed at the North American level because of the almost complete absence of the group outside this continent. Second, North American coelurosaurs, pachycephalosaurs, ceratopsids, and hadrosauroids, whose ages are better constrained than taxa from other areas [47] , [48] , were placed in three approximately equal-length temporal bins spanning the terminal 12 million years of the Cretaceous (77–74 Myr ago, 73–70 Myr ago, 68–65 Myr ago). Most terminal Cretaceous dinosaur-bearing formations can confidently be assigned either a late Campanian or Maastrichtian age, but, if not, we used a conservative approach and regarded taxa from these formations as ranging through the late Campanian and Maastrichtian (and thus they were placed in both time bins). In the three-bin approach, if taxa were known from the first and third time bin, then they were also assumed to be present in the intervening time bin. The Djadokhta Formation is here considered to be late Campanian in age and the overlying Nemegt Maastrichtian, following the latest work on Asian Late Cretaceous stratigraphy [49] , [50] . There is some uncertainty regarding whether the Nemegt is entirely Maastrichtian or if its base may be late Campanian in age. Fortunately, only one of our datasets (coelurosaurs) includes taxa from both the Djadokhta and Nemegt. In this case, our decision to regard these formations as late Campanian and Maastrichtian in age, respectively, should maximize the differences between the two time bins, making it more likely that they exhibit a significant disparity difference. However, we find no significant change in coelurosaur disparity between the late Campanian and Maastrichtian, even with this strategy. How to cite this article: Brusatte S. L. et al . Dinosaur morphological diversity and the end-Cretaceous extinction. Nat. Commun. 3:804 doi: 10.1038/ncomms1815 (2012).